Wheat powdery mildew resistance genePm13encodes a mixed lineage kinase domain-like protein Wheat powdery mildew is one of the most destructive diseases threatening global wheat production. The wild relatives of wheat constitute rich sources of diversity for powdery mildew resistance. Here, we report the map-based cloning of the powdery mildew resistance gene Pm13 from the wild wheat species Aegilops longissima . Pm13 encodes a mixed lineage kinase domain-like (MLKL) protein that contains an N-terminal-domain of MLKL (MLKL_NTD) domain in its N-terminus and a C-terminal serine/threonine kinase (STK) domain. The resistance function of Pm13 is validated by mutagenesis, gene silencing, transgenic assay, and allelic association analyses. The development of introgression lines with significantly reduced chromosome segments of Ae. longissima encompassing Pm13 enables widespread deployment of this gene into wheat cultivars. The cloning of Pm13 may provide valuable insights into the molecular mechanisms underlying Pm13 -mediated powdery mildew resistance and highlight the important roles of kinase fusion proteins (KFPs) in wheat immunity. Bread wheat ( Triticum aestivum L., 2 n = 6 x = 42) is one of the most important crops in the world and provides 20% of the total daily calories and protein for humans [1] . Wheat powdery mildew, caused by the fungus Blumeria graminis f. sp. tritici (Bgt) , is one of the most devastating diseases affecting grain yield and seed quality and can lead to an estimated yield loss-of approximately 1.07% globally [2] . The development of disease-resistant cultivars is considered the most economical and effective method for controlling this disease. A majority of the resistance (R) genes cloned to date encode nucleotide-binding domain leucine-rich repeat (NLR) immune receptors that recognize pathogen strain-specific effectors and activate effector-triggered immunity (ETI) [3] . However, race-specific resistance genes have become ineffective with the rapid evolution and emergence of new virulent isolates [4] . Recent research has shown that Triticeae contain an extended array of resistance genes that include diverse kinase domains [4] , [5] , [6] , which are new players in plant immunity. Therefore, cloning novel types of powdery mildew resistance ( Pm ) genes could facilitate their fast-tracking in breeding programs and incorporation into polygene stacks to maximize the durability of powdery mildew resistance. Although more than 60 official Pm resistance genes ( Pm1 - Pm69 ) have been identified in wheat and its wild relatives [7] , [8] , so far only 16 of these genes have been cloned and characterized. Most of these isolated Pm genes, including Pm3 [9] , Pm8 [10] , Pm2 [11] , Pm21 [12] , [13] , Pm60 [14] , Pm17 [15] , Pm41 [16] , Pm5e [17] , Pm1a [18] , MlIW172/MlWE18 [19] , Pm12 [20] and Pm69 [8] , encode NLR immune receptors. Only a few partial resistance genes have been identified, including Pm38/Yr18/Lr34/Sr57 and Pm46/Yr46/Lr67/Sr55 , which encode an ATP-binding cassette (ABC) transporter and a hexose transporter [21] , [22] , respectively. Among the recently cloned genes, Pm24 ( WTK3 ) and WTK4 encode tandem kinase proteins [4] , [6] , and Pm4 encodes a chimeric protein of a serine/threonine kinase and multiple C2 domains and transmembrane regions [5] . The genetic bottlenecks associated with wheat polyploidization and domestication, as well as selection in agroecosystems, led to a decrease in wheat genetic diversity and an increase in its vulnerability to biotic and abiotic stresses [23] . One way to improve resistance against these stresses is recruiting the adaptive potential of wild relatives of common wheat [24] . Aegilops longissima Schw. et Musch. (2 n = 2 x = 14, S l S l ) is a wild diploid species in the secondary gene pool of wheat [25] . It possesses considerable genetic diversity for improving grain protein [26] , tolerance to drought [27] and resistance to diseases [28] , [29] , [30] , [31] , [32] , [33] . Ae. longissima is also an important resource for powdery mildew resistance and several genes ( Pm13 , Pm66 , and Pm6Sl ) have been reported [28] , [31] , [32] . In addition to the dominant gene Pm13 identified on chromosome 3S l #1S from the Ae. longissima accession TL01 [28] , [29] , our previous study showed that chromosomes 3S l #2S from accession TL20 and 3S l #3S from accession TA1910 (TAM4) also confer powdery mildew resistance [30] , the resistance genes on these chromosomes were temporarily designated Pm13a and Pm13b , respectively. Furthermore, we recently introgressed Pm66 located on chromosome 4S l , and Pm6Sl located on 6S l from Ae. longissima into wheat via wheat- Ae. longissima recombination [31] , [32] . Although some of these genes ( Pm13 ) were transferred to wheat more than 30 years ago, none of those genes have been cloned to date. This limits the understanding of their molecular basis for conducting disease resistance and deployment in wheat breeding via functional molecular marker-assisted selection (MAS) or as multigene cassettes. In this work, we clone the powdery mildew resistance gene Pm13 using a strategy that combines classical map-based cloning with ph1b -induced homoeologous recombination and RNA-seq of the Pm13a donor parent TA3575 inoculated with the Bgt isolate E09. Pm13 encodes a mixed lineage kinase domain-like (MLKL) protein with an N-terminal-domain of MLKL (MLKL_NTD) domain in N-terminus and a C-terminal serine/threonine kinase (STK) domain. Pm13 orthologues are present only in the S-genome of Aegilops . Thus, cloning Pm13 will aid in elucidating the molecular mechanism of wheat powdery mildew resistance. Initial mapping of Pm13a In our previous study, Pm13a was localized on the short arm of Ae. longissima chromosome 3S l #2 in the Chinese Spring (CS)- Ae . longissima 3S l #2(3B) disomic substitution line TA3575 from accession TL20 [30] . To map the Pm13a gene, a total of 43 3S l #2-specific markers were designed based on the transcriptome sequence of the Pm13a donor parent TA3575 [34] (Supplementary Data 1 ). To induce recombination between Ae. longissima chromosome 3S l #2 and the homoeologous group 3 chromosome of common wheat, TA3575 was crossed with the CS ph1b mutant TA3809, which significantly promoted homoeologous recombination. The 300 BC 1 F 1 plants were genotyped using the ph1b -specific marker ABC302.3 [35] and two 3S l #2-specific molecular markers CL79382 and CL10208, and 25 individuals monosomic for 3S l #2 and homozygous for ph1b were selected and self-pollinated to produce BC 1 F 2 segregating populations for developing 3S l #2 recombinants. A total of 1580 BC 1 F 2 plants were screened using four 3S l #2-specific markers, which included the markers CL54397 and CL88266 at the distal ends, and the markers CL1543 and CL90315 in the proximal regions of each arm of 3S l #2. As a result, 46 plants displaying markers disassociation were selected as 3S l #2 recombinants. These 46 recombinants were further characterized using 43 3S l #2-specific markers and categorized into 22 different groups (Supplementary Data 2 ). The F 2 families of each recombinant were evaluated for powdery mildew resistance by inoculation with the Bgt isolate E09. Marker characterization of 46 3S l #2 recombinants and powdery mildew resistance evaluation resulted in physical mapping of Pm13a to the 3.67 Mb terminal interval on 3S l #2 S flanked by markers CL10208 and CL56281 (Supplementary Fig. 1 ). Seven markers (CL22345, CL87265, CL61058, CL897, CL51739, CL3352 and CL9539) were found to cosegregate with Pm13a in the mapped region (Fig. 1a, b ). Fig. 1: Map-based cloning of Pm13a. a Ae. longissima chromosome 3S l #2. b Initial mapping of Pm13a to a 3.67 Mb genomic region flanked by markers CL10208 and CL56281 on the short arm of chromosome 3S l #2. c Fine mapping of Pm13a to a 124.43 kb region between markers 3Sl-44661 and 3Sl-31B on the Ae. longissima chromosome arm 3S l #2S. d Pm13a candidate genes predicted in the 3Sl-44661-3Sl-31B marker interval. Six genes were identified in this interval, these genes, an NB-ARC domain-containing protein (NB-NRC), a cysteine-rich receptor-like protein kinase (CRK), a flavin-containing monooxygenase (FMO), an unknown protein (UN) and a protein that mediates both low-affinity uptake and efflux of sugar across the membrane (SWEET) were obtained from the Ae. longissima TL05 reference genome. A serine/threonine protein kinase (STPK) was identified from unigene CL897Contig1 in the TA3575 transcriptome sequence and was missing from the Ae. longissima TL05 reference genome. Full size image High-resolution mapping and cloning of Pm13a To fine-map Pm13a , we developed an additional set of 14 3S l #2-specific markers from recently released Ae. longissima reference sequences [36] , [37] (Supplementary Data 3 ) and used them to identify 65 3S l #2 recombinants from self-pollinated progenies of heterozygous resistant 3S l #2 recombinants (Supplementary Data 4 ). Analysis of 65 recombinants using the 14 new and seven above-mentioned markers in conjunction with the response to E09 infection resulted in the delimitation of Pm13a to a 124.43 kb interval flanked by markers 3Sl-44661 and 3Sl-31B in Ae. longissima TL05 reference genome (Supplementary Fig. 2 , Fig. 1c ). The Pm13a interval based on TL05 reference genome [36] included only five annotated genes, TL05.3S01G0012000.1, which encodes a protein with an NB-ARC domain ( NB-ARC ); TL05.3S01G0012100.1, which encodes a cysteine-rich receptor-like protein kinase ( CRK ); TL05.3S01G0012200.1, which encodes a flavin-containing monooxygenase ( FMO ); TL05.3S01G0012300.1, which encodes an unknown protein ( UN ); and TL05.3S01G0012400.1, which encodes a protein that mediates both low-affinity uptake and efflux of sugar across the membrane ( SWEET ) (Fig. 1d ). Furthermore, four markers (CL897, 3Sl-46001, 3Sl-28A and 3Sl-29B) cosegregated with Pm13a in this interval, of which only the CL897 marker, which was derived from the TA3575 transcriptome unigene CL897Contig1, was annotated as a serine/threonine protein kinase ( STPK ) (Supplementary Data 5 , Fig. 1d ) and was missing from the TL05 reference genome assembly. The remaining three markers, though present in the Ae. longissima reference sequences were not annotated as genes. Transcriptome comparison between TA3575 and CS revealed that only STPK was specifically expressed in TA3575 before and after Bgt E09 inoculation, whereas none of the five annotated genes from the TL05 reference genome were expressed in both TA3575 and CS. Sequence alignment revealed that STPK was present only in TA3575 and was absent in both CS and TL05 reference genomes. Thus, the STPK gene was considered the best candidate for Pm13a . The full-length sequence of STPK was cloned from TA3575 using the primers listed in Supplementary Data 6 . The STPK gene is 6552 bp from the start codon to the stop codon and contains seven exons with a coding sequence (CDS) of 1431 bp. The gene encodes a 476-amino acid protein containing a MLKL_NTD domain in its N-terminus and a C-terminus STK domain based on the conserved domain database from the National Center for Biotechnology Information (NCBI), which possesses the same MLKL domain architecture as the vertebrate necroptosis mediator MLKL [38] , thus STPK was re-designated as AelMLKL . Validation of AelMLKL by loss-of-function mutants To determine whether AelMLKL was required for Pm13a resistance, we mutagenized 4800 seeds of TA3575 with 0.6% ethylmethanesulfonate (EMS), and 506 M 1 plants were harvested. Sixteen M 2 seedlings from each M 1 family were screened for susceptible mutants using the Bgt isolate E09, and twenty-five families segregating for resistance and susceptibility were identified and tested in the M 3 generation. Finally, 14 independent susceptible mutants were verified after powdery mildew resistance evaluation, 3S l #2-specific marker analysis, and in situ hybridization identification in the M 3 generation. When comparing both cDNA and gDNA sequences of the AelMLKL gene from these mutants with those of TA3575, 11 out of 14 susceptible mutants had single nucleotide polymorphisms (SNPs) or deletions that resulted in amino acid substitutions, premature stop codon or frameshift mutation (Fig. 2a, b , Supplementary Fig. 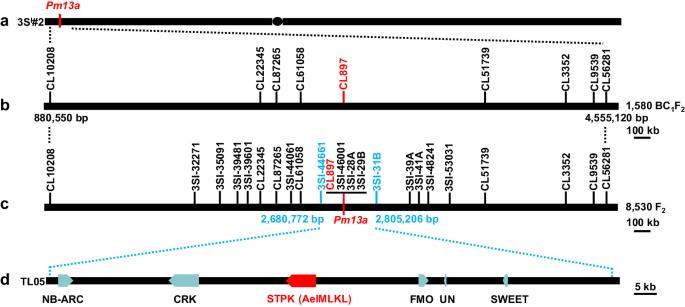Fig. 1: Map-based cloning ofPm13a. aAe. longissimachromosome 3Sl#2.bInitial mapping ofPm13ato a 3.67 Mb genomic region flanked by markers CL10208 and CL56281 on the short arm of chromosome 3Sl#2.cFine mapping ofPm13ato a 124.43 kb region between markers 3Sl-44661 and 3Sl-31B on theAe. longissimachromosome arm 3Sl#2S.dPm13acandidate genes predicted in the 3Sl-44661-3Sl-31B marker interval. Six genes were identified in this interval, these genes, an NB-ARC domain-containing protein (NB-NRC), a cysteine-rich receptor-like protein kinase (CRK), a flavin-containing monooxygenase (FMO), an unknown protein (UN) and a protein that mediates both low-affinity uptake and efflux of sugar across the membrane (SWEET) were obtained from theAe. longissimaTL05 reference genome. A serine/threonine protein kinase (STPK) was identified from unigene CL897Contig1 in the TA3575 transcriptome sequence and was missing from theAe. longissimaTL05 reference genome. 3 , Supplementary Table 1 ). Mutant F (MutF) had one missense mutation in the MLKL_NTD domain (p.G91D). MutI had a 2-bp deletion in the MLKL_NTD domain that led to a frameshift mutation. MutH had one missense mutation in the brace region between the MLKL_NTD and STK domains (p.E186K). MutK was a nonsense mutation that gave rise to premature stop codons at the encoded amino acid positions of 431 in the STK domain (p.W431*). MutA had two missense mutations within the STK domain (p.S248N and p.S371L). The remaining six independent mutants (MutB, MutC, MutD, MutE, MutG and MutJ) each had a nonsynonymous mutation (p.P395S in MutB, p.P363S in MutC, p.L310F in MutD, p.G391E in MutE, p.G332E in MutG and p.P395L in MutJ) in the STK domain. These independent mutations demonstrated that the MLKL_NTD and STK domains and the connection brace of AelMLKL are necessary for the resistance response against Bgt . No sequence variation was detected for the other three EMS-induced susceptible mutants in the AelMLKL gene, suggesting possible mutations in other unknown genes involved in the AelMLKL regulatory pathway. Fig. 2: Validation of Pm13a candidate gene AelMLKL using EMS-induced mutants and VIGS. a Powdery mildew resistance assessments of AelMLKL EMS mutants. Infection phenotypes of resistant line TA3575, susceptible control CS, and 11 susceptible mutants inoculated with Bgt isolate E09 at 7 d post-inoculation (dpi). b EMS-induced mutants carrying frameshift, nonsense, and missense mutations in the AelMLKL gene sequence. The structure of the AelMLKL gene (from the start to the stop codon) is presented. Black straight lines indicate introns, and rectangles indicate coding exons (red, magenta and bright orange rectangles represent the MLKL_NTD and STK domains, and the brace region, respectively). The positions of the mutations are indicated by thin vertical lines. Mutation names in black indicate the coding sequence (c.) changes and their predicted effects on the translated protein (p.). c Symptoms of the third leaves of representative plants subjected to VIGS at 7 days after inoculation with Bgt isolate E09 are shown. d Expression levels of the AelMLKL of BSMV:γ- and BSMV: AelMLKL- infected TA3575 plants assessed via qRT-PCR. Five leaves were used for each biological replicate, and three biological replicates were used for each group. The values of qRT-PCR are the mean ± SD (two-sided t -test, n = 3 biologically independent experiments, *** P < 0.001). Source data are provided as a Source Data file. Full size image Silencing of AelMLKL compromises powdery mildew resistance in TA3575 To further validate whether AelMLKL mediates resistance to powdery mildew, we employed Barley stripe mosaic - virus-induced gene silencing ( BSMV -VIGS) to specifically knock down the expression of the AelMLKL gene in TA3575. Powdery mildew symptoms and fungal sporulation pustules were observed on the leaves with reduced AelMLKL expression through VIGS (Fig. 2c, d ), confirming that a high level of powdery mildew resistance in TA3575 required a certain level of AelMLKL expression. Transgenic expression validates AelMLKL as Pm13a To further validate whether AelMLKL was sufficient to confer powdery mildew resistance, we performed transgenic expression via the CDS of AelMLKL driven by the maize ubiquitin ( Ubi ) promoter into susceptible wheat cultivar Fielder. As a result, 14 of the 20 transgenic T 0 plants were confirmed to have AelMLKL by PCR analysis and conducted immune responses to Bgt isolate E09 (Infection type (IT) = 0) (Fig. 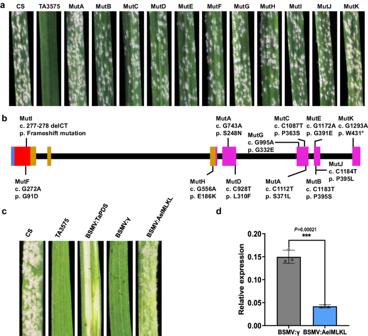Fig. 2: Validation ofPm13acandidate geneAelMLKLusing EMS-induced mutants and VIGS. aPowdery mildew resistance assessments ofAelMLKLEMS mutants. Infection phenotypes of resistant line TA3575, susceptible control CS, and 11 susceptible mutants inoculated withBgtisolate E09 at 7 d post-inoculation (dpi).bEMS-induced mutants carrying frameshift, nonsense, and missense mutations in theAelMLKLgene sequence. The structure of theAelMLKLgene (from the start to the stop codon) is presented. Black straight lines indicate introns, and rectangles indicate coding exons (red, magenta and bright orange rectangles represent the MLKL_NTD and STK domains, and the brace region, respectively). The positions of the mutations are indicated by thin vertical lines. Mutation names in black indicate the coding sequence (c.) changes and their predicted effects on the translated protein (p.).cSymptoms of the third leaves of representative plants subjected to VIGS at 7 days after inoculation withBgtisolate E09 are shown.dExpression levels of theAelMLKLof BSMV:γ- and BSMV:AelMLKL-infected TA3575 plants assessed via qRT-PCR. Five leaves were used for each biological replicate, and three biological replicates were used for each group. The values of qRT-PCR are the mean ± SD (two-sidedt-test,n= 3 biologically independent experiments, ***P< 0.001). Source data are provided as a Source Data file. 3 , Supplementary Table 2 ). Among the 14 T 1 transgenic positive plants resulting from self-pollination of different T 0 individuals, AelMLKL-OE3 displayed no significant difference in AelMLKL expression compared to TA3575, while the remaining 13 T 1 lines exhibited higher AelMLKL expression (Supplementary Fig. 4 ). These results indicated that both normal expression and overexpression of AelMLKL can effectively respond to Bgt isolate E09. Taken together, the results from the EMS mutagenesis, BSMV -VIGS, and transgenic experiments consistently support that AelMLKL is the functional Pm13a gene. Fig. 3: Transgenic validation of Pm13a candidate gene AelMLKL. a Structure of ProUbi : AelMLKL used for transformation of susceptible cultivar Fielder. The construct contains the gene coding sequence (CDS), the maize ubiquitin ( Ubi ) promoter, and nopaline synthase ( Nor ) terminator. LB left border, RB right border. b Powdery mildew responses of the resistant line TA3575 (IT 0), Fielder (IT 4), and the T 1 transgenic plants of ProUbi : AelMLKL (IT 0) to Bgt isolate E09. Three representative individuals of each transgenic line were photographed at 7 dpi; the presence (+) or absence (–) of AelMLKL is indicated. Full size image Allelism at the Pm13 locus We previously reported that Pm13 (R1B), Pm13a (TA3575), and Pm13b (TA7545) are located on the short arms of chromosome 3S l from different Ae. longissima accessions [30] . To determine whether these three genes are the same, we first performed an allelism test by conducting reciprocal crosses with R1B ( Pm13 ), TA3575 ( Pm13a ), and TA7545 ( Pm13b ), and subsequently phenotyped their F 2 individuals by inoculation with the Bgt isolate E09 at the seedling stage. 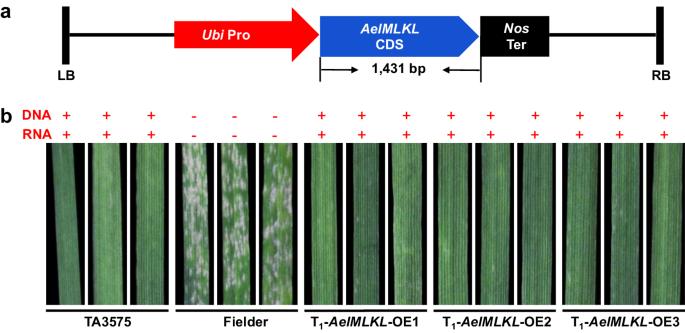Fig. 3: Transgenic validation ofPm13acandidate geneAelMLKL. aStructure ofProUbi:AelMLKLused for transformation of susceptible cultivar Fielder. The construct contains the gene coding sequence (CDS), the maize ubiquitin (Ubi) promoter, and nopaline synthase (Nor) terminator. LB left border, RB right border.bPowdery mildew responses of the resistant line TA3575 (IT 0), Fielder (IT 4), and the T1transgenic plants ofProUbi:AelMLKL(IT 0) toBgtisolate E09. Three representative individuals of each transgenic line were photographed at 7 dpi; the presence (+) or absence (–) ofAelMLKLis indicated. All the F 2 plants from the crosses R1B × TA3575 (2183 plants), R1B × TA7545 (2715 plants), TA3575 × R1B (2785 plants), TA3575 × TA7545 (2176 plants), TA7545 × R1B (2082 plants) and TA7545 × TA3575 (2168 plants) displayed no segregation for powdery mildew resistance (Supplementary Table 3 ). Furthermore, we performed a resistance spectrum assay using 36 Bgt isolates with different virulence spectra collected from the main wheat-growing provinces of China, the R1B, TA3575, and TA7545 lines were immune or highly resistant to each Bgt isolate (IT 0-1) at the seedling stage (Supplementary Data 7 ). These results proved that Pm13 , Pm13a , and Pm13b are allelic or tightly linked. Subsequently, comparing the gDNA sequences of the AelMLKL gene from these accessions confirmed that R1B and TA7545 had AelMLKL gene sequences identical to that of TA3575, thus providing strong evidence that Pm13 , Pm13a , and Pm13b are the same gene. Subcellular localization and structural analysis of the Pm13 protein To determine the subcellular location of Pm13, we fused the Pm13 gene (CDS sequence without the terminal codon) to the N-terminus of a green fluorescent protein (GFP) reporter gene, and the resulting expression cassette ( 35S::Pm13-GFP ) was transiently expressed in wheat leaf protoplasts. As shown in Supplementary Fig. 5 , green fluorescence was ubiquitously detected in the cells transformed with the 35S::GFP control. Similarly, fluorescence of the Pm13-GFP fusion protein was observed in the nucleus and cytoplasm. To understand its detailed architecture, we used AlphaFold v2.0 [39] to construct a three-dimensional (3D) model of Pm13. The 3D model revealed that the N-terminal MLKL_NTD domain of Pm13 consisted of a four-helix bundle (4HB) structure that is also defined as the HeLo domain or DUF1221 domain (Fig. 4a, b ). The C-terminal STK domain of Pm13 was composed of a smaller N-lobe made up of five antiparallel β strands and the helix αC, and a larger C-lobe composed principally of α helices (Fig. 4a, c ), and the two domains were connected by a three helices-containing brace (Fig. 4a ). The frameshift, missense, and nonsense mutations of 11 susceptible mutants spread across the MLKL_NTD and STK domains, and their brace connection of Pm13 and resulted in loss-of resistance to powdery mildew, indicating that both the domains and connection brace might be required for Pm13 to confer resistance against powdery mildew. Fig. 4: Protein structure prediction and mutation analysis of Pm13. a Tertiary structure of Pm13 predicted by AlphaFold v2.0. b MLKL_NTD domain predicted by AlphaFold v2.0; the MLKL_NTD domain consists of a four-helix bundle (4HB) structure. c STK domain predicted by AlphaFold v2.0, indicating the basic secondary functional features. Red: MLKL_NTD domain; Magenta: STK domain; Bright orange: Brace. Yellow spheres indicate internal amino acid substitutions resulting from the EMS mutagenesis. Cyan spheres represent surface-localized amino acid substitutions. Full size image Structural homology modeling of the Pm13 protein revealed that the N-terminal MLKL_NTD domain of Pm13 superimposed well with the MLKL_NTD domain of animal MLKL [38] , the DUF1221 domain of Arabidopsis thaliana AtMLKL [40] and the CC R domain of Nicotiana benthamiana NRG1.1 [41] (Supplementary Fig. 6 ). All of these domain-containing proteins are involved in regulating cell death [38] , [40] , [42] . The C-terminal kinase domain of Pm13, in contrast to the pseudokinase domains of the mammalian MLKL and A. thaliana AtMLKLs, contains all the key conserved residues for kinase activity according to sequence alignment [43] (Supplementary Data 8 ). Pm13 is predicted to be a functional protein kinase based on the presence of key residues for kinase activity. Therefore, Pm13 encodes a kinase fusion protein (KFP) with an unusual domain architecture that contains a C-terminus kinase domain fused to a MLKL_NTD domain in the N-terminus, this structure is obviously different from that of other cloned plant disease resistance genes. Phylogenetic analysis of Pm13 Mahdi et al. identified a limited number of MLKL proteins [40] , and the N-terminal domain of these MLKLs was classified as the DUF1221 domain. To investigate the evolutionary relationships between Pm13 and other MLKLs, we retrieved 714 MLKL_NTD-Kinase proteins (Supplementary Data 9 ) and 97 DUF1221-Kinase proteins (Supplementary Data 10 ) in Poaceae and Arabidopsis from the Interpro database ( https://www.ebi.ac.uk/interpro ) and conducted phylogenetic analysis together with Pm13 and three AtMLKL proteins. These 815 proteins were classified into two distinct clusters, namely, the MLKL_NTD-Kinase cluster and the DUF1221-Kinase cluster. Pm13 belonged to the MLKL_NTD-Kinase cluster but was in a subfamily distinct from any other MLKL_NTD-Kinase proteins (Supplementary Fig. 7 ). We used a Hidden Markov Model-based classification approach for protein kinases developed by Lehti-Shiu & Shiu [44] to analyze the evolution of the Pm13 kinase domain. The results showed that the Pm13 kinase domain belongs to the DLSV (DUF26, SD-1, LRR-VIII, and VWA) protein kinase subfamily in the RLK (receptor-like kinase)/Pelle family. Further investigation revealed that at least 44 proteins in Poaceae shared more than 60% sequence identity with the Pm13 kinase domain. The closest homolog of the Pm13 kinase domain was the cysteine-rich receptor-like kinase (CRK) encoded by the T. dicoccoides CRK26 gene (Supplementary Data 11 ). Phylogenetic analysis of the kinase domains of Pm13 and those 44 homologs together with recently cloned KFPs, revealed that the kinase domain of Pm13 and 44 homologs belong to the LRR_8B subfamily (Supplementary Fig. 8 ), the most frequent kinase subfamily found in cloned KFPs [45] . We performed a BLASTP search using the MLKL_NTD domain of Pm13 across the Triticeae tribe in WheatOmics ( http://wheatomics.sdau.edu.cn/ ), which identified 220 MLKL_NTD domain-containing proteins (Supplementary Data 12 , 13 ) and 228 MLKL_NTD domains (Supplementary Data 14 ). The phylogenetic trees revealed that Pm13 and three MLKL_NTD-Kinase proteins from the S-genome of Aegilops species were in the same clade (Supplementary Figs. 9 , 10 ). Among them, TB01.3S01G0016800.1 from Ae. bicornis TB01, TH02.3S01G0013600.2 from Ae. sharonensis TH02 and TS01.3B01G0036300.1 from Ae . 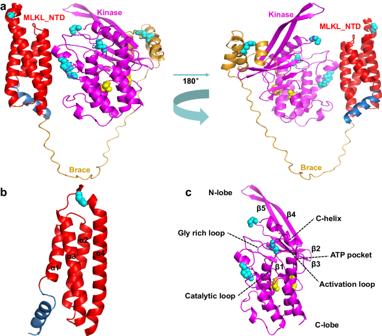Fig. 4: Protein structure prediction and mutation analysis of Pm13. aTertiary structure of Pm13 predicted by AlphaFold v2.0.bMLKL_NTD domain predicted by AlphaFold v2.0; the MLKL_NTD domain consists of a four-helix bundle (4HB) structure.cSTK domain predicted by AlphaFold v2.0, indicating the basic secondary functional features. Red: MLKL_NTD domain; Magenta: STK domain; Bright orange: Brace. Yellow spheres indicate internal amino acid substitutions resulting from the EMS mutagenesis. Cyan spheres represent surface-localized amino acid substitutions. 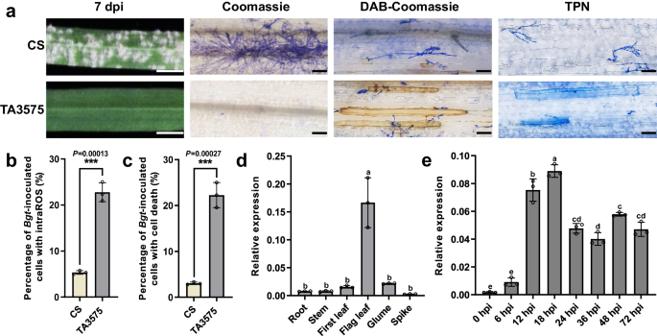Fig. 5: Phenotype and expression patterns ofPm13afterBgtinoculation. aMacroscopic and microscopic characterization of TA3575 and the susceptible control CS after inoculation withBgtisolate E09. From left to right: Macroscopic view of the infected leaf segments at 7 dpi. Scale bar, 5 mm. Coomassie blue staining of infected leaves at 7 dpi to visualize fungal structures. Bar, 10 μm. DAB-Coomassie blue staining of infected leaves at 48 hpi. Brown staining showed ROS accumulation. Bar, 10 μm. Trypan blue staining of the infected leaves at 48 hpi to visualize cell death. Bar, 10 μm.bPercentage ofBgt-inoculated cells with intraROS. The values are the mean ± SD (two-sidedt-test,n= 3 biologically independent experiments, ***P< 0.001).cPercentage of cells with cell death ofBgt-inoculated cells. The values are the mean ± SD (two-sidedt-test,n= 3 biologically independent experiments, ***P< 0.001).dTranscript levels ofPm13in different tissues of TA3575, including the first leaves at three-leaf stage and roots, stems, flag leaves, glumes, and spikes at the heading stage, determined via qRT-PCR. The values of qRT-PCR are the mean ± SD (one-way ANOVA with Tukey’s test,n= 3 biologically independent experiments).eqRT-PCR analysis ofPm13expression in one-week-old TA3575 seedings at 0, 6, 12, 18, 24, 36, 48, and 72 hpi with theBgtisolate E09. The expression of the genes was evaluated via qRT-PCR, withTaActinserving as an endogenous control, and the expression was calculated using the comparative CT method. The values of qRT-PCR are the mean ± SD (one-way ANOVA with Tukey’s test,n= 3 biologically independent experiments). Source data are provided as a Source Data file. speltoides TS01 shared 99.37%, 97.27%, and 89.94% protein sequence identity with Pm13, respectively (Supplementary Table 4 , Supplementary Fig. 11 ). Further synteny analysis using five Ae. longissima genes on either side of Pm13 across the Triticeae tribe demonstrated that these three genes were orthologous to Pm13 (Supplementary Fig. 12 ). These findings suggest that the Pm13 architecture may be present only in the S-genome of the Aegilops genus and that the Pm13 gene may have arisen after the origin of the S-genome. Expression pattern of Pm13 We visualized the resistance phenotype of Pm13 with leaves infected with the Bgt isolate E09 at 7 d post-inoculation (dpi). TA3575 was highly resistant to Bgt isolate E09, with no visible conidia produced (IT 0), while CS was highly susceptible, with a large number of visible conidia (IT 4). DAB and Trypan blue staining showed higher intracellular reactive oxygen species (intraROS) levels and greater cell death in TA3575 compared to CS (Fig. 5a–c ). Quantitative RT-PCR (qRT-PCR) analysis revealed that the expression of Pm13 was highest in flag leaves (Fig. 5d ), with expression upregulated with a slight increase at 6 h post-inoculation (hpi), peaking at 12–18 hpi, and decreasing thereafter (Fig. 5e ). Fig. 5: Phenotype and expression patterns of Pm13 after Bgt inoculation. a Macroscopic and microscopic characterization of TA3575 and the susceptible control CS after inoculation with Bgt isolate E09. From left to right: Macroscopic view of the infected leaf segments at 7 dpi. Scale bar, 5 mm. Coomassie blue staining of infected leaves at 7 dpi to visualize fungal structures. Bar, 10 μm. DAB-Coomassie blue staining of infected leaves at 48 hpi. Brown staining showed ROS accumulation. Bar, 10 μm. Trypan blue staining of the infected leaves at 48 hpi to visualize cell death. Bar, 10 μm. b Percentage of Bgt -inoculated cells with intraROS. The values are the mean ± SD (two-sided t -test, n = 3 biologically independent experiments, *** P < 0.001). c Percentage of cells with cell death of Bgt -inoculated cells. The values are the mean ± SD (two-sided t -test, n = 3 biologically independent experiments, *** P < 0.001). d Transcript levels of Pm13 in different tissues of TA3575, including the first leaves at three-leaf stage and roots, stems, flag leaves, glumes, and spikes at the heading stage, determined via qRT-PCR. The values of qRT-PCR are the mean ± SD (one-way ANOVA with Tukey’s test, n = 3 biologically independent experiments). e qRT-PCR analysis of Pm13 expression in one-week-old TA3575 seedings at 0, 6, 12, 18, 24, 36, 48, and 72 hpi with the Bgt isolate E09. The expression of the genes was evaluated via qRT-PCR, with TaActin serving as an endogenous control, and the expression was calculated using the comparative CT method. The values of qRT-PCR are the mean ± SD (one-way ANOVA with Tukey’s test, n = 3 biologically independent experiments). Source data are provided as a Source Data file. Full size image To evaluate the impact of Pm13 on the expression of pathogenesis-related ( PR ) genes involved in plant defense, we assessed the transcript levels of six PR genes ( PR1 , PR2 , PR3 , PR4 , PR5, and PR9 ) in Pm13 transgenic lines and the susceptible control Fielder at different time points after inoculation with the Bgt isolate E09. Prior to infection, both the Pm13 transgenic lines and the susceptible control Fielder presented relatively low levels of PR gene transcripts. After inoculation, the transcript levels of the PR genes increased in both the Pm13 transgenic lines and the susceptible control Fielder, however, the Pm13 transgenic lines exhibited significantly greater transcript levels of the PR genes than did the susceptible control Fielder (Supplementary Fig. 13 ). This indicated that fungal effectors probably suppressed the expression of the PR genes in the susceptible control Fielder. Development of diagnostic markers and desirable introgression line for Pm13 The Pm13 sequence was used to develop two functional markers, AelMLKL-1 and AelMLKL-8 (Supplementary Data 6 ), that were uniquely amplified in Pm13 stocks but were absent in 180 wheat lines lacking Pm13 (Supplementary Data 15 , Supplementary Fig. 14 ). Furthermore, we developed a T3S l #2S-3BS.3BL recombinant W12-3 (Supplementary Data 4 ), which has a small 3S l #2 segment harboring Pm13 in wheat background, the Ae. longissima 3S l chromosome segment length in the recombinant wheat chromosome was estimated to be approximately 2.82 Mb based on the Ae. longissima TL05 reference genome, which will likely minimize linkage drag. The recombinant W12-3 and diagnostic markers of Pm13 will facilitate effective deployment of Pm13 in elite wheat varieties across the world. Over the past 100 years, the bread wheat gene pool has been endowed with 198 exotic resistance (R) genes, constituting 42% of the total 467 R genes designated in wheat [46] . Approximately 81 Triticeae resistance genes have been cloned to date, of which the common classes encoded NLRs [47] . Recently, resistance genes encoding KFPs have expanded the repertoire of non-NLR genes in the Triticeae tribe for resistance breeding [48] . Here, we report the map-based cloning of the wheat powdery mildew resistance gene Pm13 and confirm that AelMLKL is the causal gene by gain-of-resistance via gene transfer to a susceptible hexaploid wheat variety and suppression and loss-of-resistance through VIGS and EMS mutants. Pm13 encodes a KFP that contains a kinase domain in its C-terminus fused to the MLKL_NTD domain in the N-terminus, an unusual domain architecture compared to other cloned KFPs (such as Rpg1 [49] , Yr15 [50] , Sr60 [51] , Sr62 [52] , Pm24 [4] , WTK4 [6] , Rwt4 [53] , Yr 36 [54] , Pm4 [5] , Snn3 [55] , Tsn1 [56] , Rpg5 [57] , Sm1 [58] , Lr9 [59] , and Sr43 [47] ). KFPs have one apparent functional kinase domain that is fused to a second typically non-functional kinase domain or an entirely different domain. The integrated domains in KFPs were hypothesized to perceive pathogen effectors, while the kinase catalyzes the phosphorylation of either the effector or the NLR guard to initiate downstream defense responses and immunity [47] , [48] , [59] . Evidence for this model is provided by studies of plant NLRs with integrated domains [48] , [60] , [61] . Unlike the C-terminal pseudokinase domain of animal MLKLs and plant AtMLKLs, the C-terminal kinase domain of Pm13 comprises conserved residues crucial for kinase activity, as evidenced by sequence alignment [43] . The resistance loss induced by nine mutant sites from eight mutants located in the kinase domain of Pm13 suggested that the kinase domain is essential for Pm13-mediated activation of immune responses (Fig. 2a, b ). Nonetheless, whether the C-terminal kinase domain of Pm13 can trigger downstream defense responses and immune reactions has yet to be proven. The Pm13 domain architecture resembled that of mammalian MLKL, which has an N-terminal MLKL_NTD domain and a C-terminal STK domain. The N-terminal MLKL_NTD domain of Pm13 is strikingly similar to the cell death-inducing HeLo and CC R domains in animals, plants, and fungi [38] , [40] , [41] , [42] , [62] . The N-terminus HeLo domain-containing MLKL protein can mediate necroptosis in animals [38] . In plants, the AtMLKLs HeLo domain can elicit cell death [40] . The CC R domain present in the RPW8 and ADR1 proteins from A. thaliana and the NRG1 protein from N. benthamiana , structurally resemble the HeLo domain and have been proven to trigger cell death by disrupting membrane integrity [41] , [42] , [63] , [64] . In fungi, the HeLo domain of HET-S from Podospora anserina was also reported to be a membrane-targeting cell death-inducing domain [62] , [65] . Regulated cell death is intimately connected with innate immunity [40] . Recent studies revealed that a notable similarity of several proteins involved in regulating cell death in different kingdoms is the HeLo domain [38] , [40] , [42] , [62] . Trypan blue staining of the leaves of the Pm13 line TA3575 post Bgt isolate E09 infection revealed strong cell death (Fig. 5a, c ), which was in accordance with the findings of Li et al. [66] . It is proposed that the N-terminal MLKL_NTD domain of Pm13 may induce cell death and trigger immune signaling. However, it is paradoxical that the functions of the integrated domains fused to kinases in KFPs are presumed to involve the perception of pathogen effectors. Therefore, it is necessary to carry out experiments to determine whether the N-terminal MLKL_NTD domain of Pm13, a member of KFPs family, functions in regulating cell death like other MLKLs or perceiving pathogen effectors like other KFPs. Ae. longissima is a wild diploid species of common wheat that harbors considerable genetic diversity for wheat improvement. To data, several disease resistance genes, including Pm13 , Pm66 , and Pm6Sl , have been introgressed from Ae. longissima into wheat through the development of wheat- Ae. longissima recombinants [29] , [30] , [31] , [32] . However, no genes for resistance to any biotic or abiotic stresses have been cloned from Ae. longissima , which hinders the elucidation of the molecular mechanisms underlying these genes. Recently, the emergence of technologies based on the integration of sequencing and mutagenesis has facilitated the cloning of disease-resistance genes in wheat and its wild relatives. Mutagenesis combined with NLR gene sequencing (MutRenSeq) or chromosome sequencing (MutChromSeq) allowed rapid cloning of the resistance genes Sr22 [67] , Sr45 [67] , Sr26 [68] , Sr61 [68] , Yr5 [69] , Yr7 [69] , Pm2 [11] , Rph1 [70] , and Sr43 [47] . Mutagenesis combined with mapping and RNA-Seq (MutRNA-Seq) or isoform sequencing (MutIsoSeq) facilitated the cloning of Sr62 [52] , Lr9/Lr58 [59] , YrNAM [71] and Lr47 [72] . Long-read genome sequencing facilitated the cloning of Yr27 [73] and Pm69 [8] . Here, we report the cloning of the powdery mildew resistance gene Pm13 using a combination of ph1b -induced recombination and transcriptome sequencing of its direct donor parent TA3575. As a comparison, fine-mapping disease resistance genes such as Pm13 , which have been introgressed into common wheat from distant wheat wild relatives such as Ae. longissima , is relatively tedious due to the low exchange and recombination suppression between the alien chromatin and wheat homoeologous counterpart, which is strictly controlled by a complex Ph system in hexaploid wheat genetic backgrounds. Nonetheless, the deletion mutant of the Ph1 locus ( ph1b ) at CS 5BL can significantly increase meiotic homoeologous recombination [74] and thus has been widely used to induce wheat-alien homoeologous recombination. Homoeologous recombination induced by ph1b is beneficial not only for the map-based cloning of resistance genes that were introgressed into common wheat from its wild relatives but also for the development of introgression lines with shortened alien segments harboring resistance genes for direct use in breeding programs. In this study, a total of 111 wheat- Ae. longissima 3S l #2 recombinants were developed based on ph1b -induced homoeologous recombination and were genotyped and phenotyped to physically fine-map Pm13 to a 124.43 kb genomic region on the Ae. longissima TL05 reference sequence. Moreover, a resistant introgression line harboring Pm13 with a 2.82 Mb 3S l #2 genomic length was developed, providing an opportunity for both cloning and utilizing this resistance gene from a wild relative of wheat. In the recent past, the availability of annotated genomes of a few wild wheat plants along with the genome sequences of more than 14 hexaploid or tetraploid wheat accessions has greatly facilitated the map-based cloning of disease resistance genes in wheat [36] , [37] , [52] , [75] , [76] , [77] , [78] , [79] . However, due to large sequence differences among different accessions within the same species, the availability of one reference genome sequence sometimes hinders the ability to identify functional genes in different accessions of the same species or related species [14] , [16] . In the present study, the Pm13 genomic sequence from the Ae. longissima accession TL20 was not found in the Ae. longissima reference genome of accession TL05. To overcome this constraint, we combined physical mapping of Pm13a and transcriptome sequencing of its direct donor parent TA3575 to successfully discover that CL897Contig1 is a serine/threonine protein kinase from the TA3575 transcriptome, which was further confirmed to be Pm13a . Recently, Zou et al. reported sequence differences around the Pm60 locus in the donor parent T. urartu accession PI428309 corresponding to the reference genome sequence of T. urartu accession G1812 [14] , limiting progress in characterizing of this locus using a reference genome sequence. Under these circumstances, our study showed that transcriptome sequencing of direct donor of target genes may help avoid potential problems caused by genomic differences in the reference genome or incomplete reference genome assemblies. Thus, combining ph1b -induced recombination for fine-mapping and RNA-Seq of direct donors of target genes is a powerful tool for isolating resistance genes that have been introgressed into the hexaploid wheat background from wild species. Pm13 , located on the short arm of chromosome 3S l #1 (3S l #1S) of the Ae. longissima accession TL01 was subsequently transferred into wheat in 1988 via the induction of CS- Ae. longissima T3S l #1S-3BS.3BL and T3S l #1S-3DS.3DL recombinants [28] . The gene has maintained its effectiveness against different Bgt biotypes for more than 30 years across several countries [29] , [80] . However, the deployment of this gene has been limited in wheat breeding programs due to linkage drag, which results in inferior agronomic characteristics owing to the presence of a larger chromosomal segment of Ae. longissima [81] . In the present study, we developed a resistant T3S l #2S-3BS.3BL recombinant W12-3 strain that carried Ae. longissima segments harboring Pm13 as short as <0.35% of the 3S l #2 genomic length. This resistant introgression line could minimize the undesirable linkages associated with Pm13 . Furthermore, we designed two functional markers, AelMLKL-1 and AelMLKL-8, from Pm13 for precise marker-assisted selection of common wheat lines harboring Pm13 . The W12-3 line and two Pm13 functional molecular markers will facilitate effective wide-scale deployment of Pm13 in elite wheat varieties. In summary, we cloned the wheat powdery mildew resistance gene Pm13 from Ae. longissima . Pm13 encodes a MLKL protein that contains a MLKL_NTD domain in N-terminal and a STK domain in its C-terminus. Isolation of Pm13 will shed light on its disease resistance mechanism. In addition, the resistance introgression line harboring Pm13 within approximately 2.82 Mb of the 3S l #2 genomic length (estimated using Ae. longissima TL05 reference genome) and the developed diagnostic functional markers AelMLKL-1 and AelMLKL-8 for Pm13 will facilitate deployment of this gene in elite wheat varieties through MAS or by engineering gene pyramids that may maximize its longevity in powdery mildew resistance. Plant materials The CS- Ae. longissima recombinant lines T3S l #1S-3BS.3BL (R1B) and T3S l #1S-3DS.3DL (R2B) harboring Pm13 were developed by Ceoloni et al. [28] and provided by Nanjing Agricultural University, China. The CS- Ae. longissima 3S l #2(3B) disomic substitution line TA3575, the CS- Ae. longissima 3S l #3S isochromosome addition line TA7545, the wheat landrace CS, the CS ph1b mutant TA3809 which lacked the Ph1 gene and thereby elevated homoeologous recombination, and the Ae. longissima accession TA1910 (TAM4) were kindly provided by the Wheat Genetics Resource Center at Kansas State University, USA, and maintained at the Experimental Station of Henan Agricultural University, China. The donors of chromosomes 3S l #1 in R1B, 3S l #2 in TA3575, and 3S l #3 in TA7545 were derived accordingly from the Ae . longissima accessions TL01, TL20 and TA1910 (TAM4) [82] , [83] , [84] . The powdery mildew-susceptible wheat cultivar Fielder was used for the transformation of Pm13 . One hundred and eighty wheat lines (Supplementary Data 15 ) were used for verifying diagnostic markers for Pm13 . The plants were grown in a greenhouse with 14 h light/10 h dark (22/18 °C, 70% relative humidity). Powdery mildew resistance phenotyping Bgt isolate E09 and another 35 isolates with different virulent spectrums from different provinces of China (Supplementary Data 7 ) were used to evaluate powdery mildew resistance under controlled conditions. Bgt isolates were maintained and increased on the highly susceptible CS seedlings. Wheat seedlings at the first-leaf stage (one-week-old) were inoculated with Bgt isolates and then grew in a greenhouse at 22 °C under a 14 h light/10 h darkness photoperiod [30] . Ten individual plants for each of R1B, TA3575, TA7545, and CS were inoculated with 36 Bgt isolates. At least 16 individuals of F 2 progenies from each 3S l #2 recombinant, M 2, and M 3 families of EMS-treated mutants and transgenic families were inoculated with Bgt isolate E09 to evaluate resistance phenotypes. Infection types (ITs) were assessed at 7 dpi using a scale from 0 to 4 [85] . The phenotypes were divided into two categories, resistant (R, IT 0-2) and susceptible (S, IT 3-4). To visualize the fungal structures, the first leaves of TA3575 and CS were cut into 2 cm segments at 7 dpi with Bgt isolate E09 and fixed in a fixative (ethanol:glacial acetic acid, 3:1, v/v) for 12–16 h. Then tissue was rinsed with deionized water twice and stained with Coomassie brilliant blue (0.05% Coomassie brilliant blue R250, 10% acetic acid, 50% methanol) for 10–15 min [86] . The treated leaves were observed under the Olympus BX51 microscope (Olympus Corporation, Tokyo, Japan). Detection of ROS accumulation and plant cell death To detect the ROS accumulation, the first leaves were cut from seedlings of TA3575 and CS at 48 hpi with Bgt isolate E09 and immediately incubated in a 3,3′-diaminobenzidine (DAB) solution (1 mg/mL, pH 5.8) for 12 h, and then bleached in destaining solution (ethanol:acetic acid, 1:1, v/v) for 12–16 h. The bleached leaves were stained with 0.6% (w/v) Coomassie blue solution for 10 s and then washed with water for assessing the ROS accumulation [87] . To detect plant cell death, the first leaves from TA3575 and CS plants at 48 hpi with Bgt isolate E09 were incubated in a 0.4% Trypan blue solution for 2 min in boiling water, then bleached in chloral hydrate solution (2.5:1, w/v) for 24 h. The bleached leaves were incubated in 0.6% (w/v) Coomassie blue solution for 10 s [88] . ROS-induced epidermal cell death was observed under an Olympus BX51 microscope (Olympus Corporation, Tokyo, Japan). All microscopic experiments were conducted with three biological replicates, and at least 100 infected cells were observed for each replicate to determine ROS accumulation and cell death responses. The quantitative assessment of ROS accumulation and associated cell death was performed [66] . Initial mapping of Pm13a using CS ph1b mutant To develop 3S l #2 recombinants, the CS- Ae. longissima 3S l #2(3B) disomic substitution line TA3575 was crossed with the CS ph1b mutant TA3809. The derived BC 1 F 1 populations were screened to identify individuals homozygous for ph1b and monosomic for 3S l #2 using ph1b -specific marker ABC302.3 designed by Wang et al. [35] and 3S l #2-specific markers developed in this study. The 1580 selected individuals-derived BC 1 F 2 progenies were analyzed by four 3S l #2-specific markers (CL54397, CL1543, CL90315, and CL88266) in the distal and proximal regions of each arm of chromosome 3S l #2 to select CS- Ae. longissima 3S l #2 recombinants missing one to three markers. The recombinants were further characterized using other 3S l #2-specific molecular makers. The recombinants and derived progenies were phenotyped for resistance to the Bgt isolate E09 for initial mapping of Pm13a . All information for the 3S l #2-specific markers is listed in Supplementary Data 1 . PCR was performed in 15.0 µL volumes containing 2.0 µL template gDNA (100 ng/µL), 1.0 µL of each primer (5.0 µmol/L), 7.5 µL 2 × Es Taq MasterMix (CWBIO, Beijing, China) and 3.5 µL ddH 2 O. The PCR program consisted of initial denaturation at 95 °C for 5 min followed by 35 cycles of 95 °C for 30 s, 53–66 °C annealing for 30 s depending on different primers, and 72 °C for 1 min, with a final extension at 72 °C for 10 min. To obtain sequence polymorphisms, the PCR products without polymorphism were digested with restriction enzymes Mse I, Msp I, Mbo I, Alu I, and Rsa I (New England Biolabs, Beijing, China). Five microlitres of a restriction enzyme mixture containing 2.85 µL of ddH 2 O, 2.0 µL of CutSmart buffer, and 0.15 µL of an enzyme stock solution was added to 15.0 µL of PCR products and incubated for 3.5 h at 37 °C. The PCR or restricted PCR products were separated via gel-electrophoresis on a 2.0% agarose gel stained with ethidium bromide and visualized by UV light. High-resolution mapping of Pm13a For fine mapping of Pm13a , 8530 F 2 individuals derived from heterozygous 3S l #2 resistant recombinants were phenotyped for powdery mildew resistance and genotyped with Pm13a -flanking markers CL10208 and CL56281 to develop 3S l #2 recombinant population for high-resolution mapping in the Pm13a interval. The Ae. longissima genome sequence [36] , [37] was used to design additional markers in the mapping interval. The markers that cosegregated with Pm13a in the initial map interval were also subjected to fine-mapping. The Pm13a gene was physically fine-mapped by combining genotypic and phenotypic data for all the recombinants. RNA-Seq of Pm13a donor parent TA3575 Transcriptome sequencing of the Pm13a donor parent TA3575 and recipient parent CS was described as Dong et al. [34] . In brief, TA3575 and CS were inoculated with the Bgt isolate E09 when the first leaves were fully unfold. Leaves at 0, 12, 24, 48, and 72 hpi were respectively collected and immediately frozen in liquid nitrogen for RNA extraction. Total RNA was extracted from ten samples (0, 12, 24, 48, and 72 hpi for TA3575 and CS, respectively) for RNA-seq at OE Biotech (Shanghai, China). Then, equal amounts of RNA from TA3575 and CS at 12–72 hpi were mixed to generate RNA-seq samples TA3575_I and CS_I, respectively. RNA at 0 hpi from TA3575 and CS was accordingly represented as RNA-seq samples TA3575_C and CS_C. Two biological replicates were performed, forming a total of eight RNA samples (TA3575_I1, TA3575_I2, TA3575_C1, TA3575_C2, CS_I1, CS_I2, CS_C1, and CS_C2). Designations 1 and 2 are used to represent replicates 1 and 2, respectively. Cloning of full-length CDS of AelMLKL gene Total RNA was extracted from the E09-inoculated leaf tissue of the resistant line TA3575 using RNA isolater Total RNA Extraction Reagent (Vazyme, Nanjing, China). Reverse transcription was performed using HiScript III 1st Strand cDNA Synthesis Kit (+gDNA wiper) (Vazyme, Nanjing, China) following the manufacturer’s instructions. The full-length CDS of the AelMLKL gene was amplified using 2 × Phanta Flash MasterMix (Dye Plus) (Vazyme, Nanjing, China) by PCR with the gene-specific primer AelMLKL_CDS (Supplementary Data 6 ). The PCR product was cloned into the One step ZTOPO-Blunt/TA vector (ZOMANBIO, Beijing, China). The inserted fragment in the ZTOPO-Blunt/TA-AelMLKL_CDS construct was verified by Sanger sequencing at Sangon Biotech, Shanghai, China. EMS mutagenesis and mutant validation Seeds of TA3575 were treated with EMS as described by Ma et al. [89] . Specifically, a total of 4800 seeds were soaked in distilled water for 6 h and treated with 0.6% EMS solution on a shaker at 150 rpm for 14 h. M 0 seeds were sown in the field with 80 seeds per 2 meter-length row, and 506 M 1 plants were harvested. Sixteen M 2 seedlings from each M 1 line were inoculated with Bgt isolate E09 under controlled greenhouse conditions to identify susceptible mutants. The M 3 progenies derived from susceptible M 2 mutants were challenged again with Bgt isolate E09 to confirm their susceptibility and select homozygous mutants. The M 3 mutant lines were further validated by 3S l #2-specific markers, genomic in situ hybridization (GISH), and fluorescence in situ hybridization (FISH) analyses. The gDNA and full-length CDS of the AelMLKL gene were amplified from each of the M 3 homozygous mutants using the primers listed in Supplementary Data 6 . The PCR products were sequenced at Sangon Biotech, Shanghai, China. The AelMLKL gene sequences from the mutants and wild-type TA3575 were compared using DNAMAN 8 software (Lynnon Biosoft, San Ramon, CA, USA) to identify SNPs. Cytogenetic analyses GISH and FISH was used to rule out EMS-induced M 2 susceptible plants caused by seed contamination or loss-of 3S l #2 chromosomes and verify loss-of-function mutants. Chromosome spreads of root tip cells at mitotic metaphase were prepared following Huang et al. [90] . Root tips were exposed in an N 2 O gas chamber for 2 h followed by a 30-min treatment with 90% acetic acid. Subsequently, the root tips were rinsed three times with 75% ethanol and fixed in a fixative (ethanol:glacial acetic acid, 3:1, v/v) for 2–7 days. For GISH, total gDNA of Ae. longissima accession TL20 was labeled with fluorescein-12-dUTP and used as the probe, and unlabeled gDNA of common wheat CS was served as blocking [30] . The ratio of gDNA of Ae. longissima to CS was 1:130. After GISH, the hybridization signals were washed with phosphate-bufered saline (PBS) to conduct dual-color FISH using eight single-strand oligonucleotides pSc119.2-1, (GAA) 10 , pAs1-1, pAs1-3, pAs1-4, pAs1-6, AFA-3 and AFA-4 as probes [90] , [91] . The first two oligonucleotides were modified with 6-carboxyfuorescein (FAM), and the last six oligonucleotides were modified with 6-carboxytetramethylrhodamine (TAMRA) at the 5’-ends. Fluorescent images were captured with AxioCam MRc5 CCD camera using a Zeiss Axio Scope A1 fuorescence microscope (Germany). Images were processed using Photoshop CS 3.0 (Version 10.0.1). The oligo probes were synthesized with 5’-ends labeled with TAMRA or FAM by Sangon Biotech, Shanghai, China. Virus-induced gene silencing BSMV-VIGS was used to investigate the functions of the AelMLKL gene in TA3575 as described by Xing et al. [12] . In brief, a 246-bp target fragment with little homology (identity <50%, stretches of 100% nucleotide identity <21-nt) in the wheat assemblies was inversely inserted into the γ-strain of BSMV by replacing the TaPDS sequence of the BSMV: TaPDSas vector for construction of the BSMV: AelMLKL as recombinant silencing vector. Plasmid linearization, in vitro transcription, and virus inoculation were performed as described by Wang et al. [92] . In particular, the first fully expanded leaves of TA3575 seedlings were infected with the in vitro-transcribed BSMV: AelMLKL as virus, BSMV: TaPDSas and BSMV:γ served as controls. At 14 d after virus infection, when viral infection symptoms were clearly visible, the third leaves were detached and placed on 1% agar plates supplemented with 20 mg/mL 6-phenyladenine (6-BA). Then, the detached leaves were infected with the fresh Bgt isolate E09 and incubated at 24 °C under a 14-h light /10-h dark photoperiod with 70% humidity. After 7 days inoculation, powdery mildew disease phenotypes were evaluated and leaf samples were collected for further gene silencing expression analyses of AelMLKL . At least 15 plants were challenged by BSMV vector, and the experiments were repeated three times. Plant genetic transformation The CDS of AelMLKL flanked by a Bam HI restriction site was amplified via PCR from the ZTOPO-Blunt/TA-AelMLKL_CDS construct using the primer set AelMLKL_OETrans and cloned into the Bam HI site of the pWMB110 vector downstream of the maize ( Zea mays L.) ubiquitin ( Ubi ) promoter with the nopaline synthase ( Nor ) terminator via the ClonExpress II One Step Cloning Kit (Vazyme, Nanjing, China) to generate the overexpression vector ProUbi : AelMLKL . The colonies were sequenced to confirm the accuracy of the cDNA insertions. The ProUbi : AelMLKL plasmid was transformed into the Agrobacterium tumefaciens strain EHA105 and transformed into the susceptible wheat cultivar Fielder. Specific marker AelMLKL_OE was used to detect the presence of AelMLKL genes in the transgenic progenies. PCR primer pair AelMLKL_Exp was used to detect the expression of AelMLKL in the transgenic plants. All the primers used are listed in Supplementary Data 6 . Sixteen T 1 transgenic plants (first-leaf stage) for each transgenic event were tested for their responses to Bgt isolate E09, and disease symptoms were recorded at 7 dpi. Gene expression analysis Total RNA was extracted from the first leaves of the Pm13 transgenic lines AelMLKL-OE11 and AelMLKL-OE14, and susceptible control Fielder at the first-leaf stage before inoculation (0 hpi) and 12, 18, 24, 36, and 48 hpi with Bgt isolate E09 using TRIzol reagent (Vazyme, Nanjing, China). Each time point was composed of three biological replicates with five individuals per replicate. Reverse transcription was performed using HiScript III RT SuperMix for qPCR (+gDNA wiper) (Vazyme, Nanjing, China). qRT-PCR analysis was carried out using SYBR Mix (TaKaRa, Dalian, China) following the manufacturer’s instructions. The primers used to evaluate the transcript levels of the gene AelMLKL and PRs are listed in Supplementary Data 6 . The wheat TaActin gene was used as the endogenous control [4] . The comparative CT method was used to quantify relative gene expression [93] . For validation of VIGS, three biological replicates with five leaves per replicate were used for expression analysis. Allelism at the Pm13 locus To test the allelism of Pm13 , Pm13a , and Pm13b , reciprocal crosses were made with R1B ( Pm13 ), TA3575 ( Pm13a ), and TA7545 ( Pm13b ). All the F 2 plants derived from the crosses R1B × TA3575 (2183 plants), R1B × TA7545 (2715 plants), TA3575 × R1B (2785 plants), TA3575 × TA7545 (2176 plants), TA7545 × R1B (2082 plants) and TA7545 × TA3575 (2,168 plants) were phenotyped by inoculation of Bgt isolate E09 to investigate the segregation for powdery mildew resistance. Furthermore, the resistance spectrum of R1B, TA3575, and TA7545 were also assayed using 36 Bgt isolates with different virulent spectrum collected from the main wheat-growing provinces of China. To further test whether the Pm13 , Pm13a, and Pm13b genes are identical, the 6552 bp genomic sequences of AelMLKL gene were obtained from R1B ( Pm13 ) and TA7545 ( Pm13b ) using the primers listed in Supplementary Data 6 . The 15 µL DNA amplification system contained 7.5 µL 2 × Es Taq MasterMix (CWBIO, Beijing, China), 2.0 µL template gDNA (100 ng/µL), 1.0 µL of each primer (5.0 µmol/L) and 3.5 µL ddH 2 O. DNA amplification was performed at 95 °C for 5 min followed by 35 cycles of 95 °C for 30 s, 50–60 °C (depending on specific primers) for 30 s, and 72 °C for 1 min, with a final extension at 72 °C for 10 min. The PCR products were sequenced by Sanger dye-terminator method at Sangon Biotech, Shanghai, China. The sequences of the AelMLKL gene from R1B ( Pm13 ) and TA7545 ( Pm13b ) were compared with that from TA3575 using DNAMAN 8 software (Lynnon Biosoft, San Ramon, CA, USA). Subcellular localization analysis To determine the subcellular location of Pm13, the Pm13 coding sequence was cloned and inserted into the pJIT163-GFP vector between Hin dIII and Eco RI sites for Pm13-GFP fusion expression driven by the CaMV35S promoter ( 35S::Pm13-GFP ) in wheat protoplasts. The 35S::Pm13-GFP was cotransfected into protoplasts with the nucleus marker plasmid AtPIF4-mCherry using polyethyleneglycol (PEG)-calcium-mediated transfection [94] , [95] . The transformed protoplasts were cultured at 25 °C for 16 h under dark conditions, and observed using a laser scanning confocal microscope (A1HD25Nikon, Tokyo, Japan). Image acquisition was conducted with NIS-Elements Viewer Imaging Software (version 5.21.00). The subcellular localization of Pm13 protein was determined for three times. Protein sequence and domain analysis Prediction of the core domain of AelMLKL was performed based on the conserved domain database from the NCBI . Three-dimensional structure modeling of AelMLKL was performed using the open source code of AlphaFold v2.0 [39] with the amino acid sequence of AelMLKL as input. The output consisted of five ranked models in.pdb format. We utilized the rank_1.pdb model that contains the best predicted local distance difference test (pLDDT) score at 78.8. The 3D structural graphics were generated using PyMOL (v.2.6.0a0). Substituted residues that did not exhibit any visual surface on the 3D model were characterized as internal residues following Wang et al. [59] . Phylogenetic analysis of Pm13 We first retrieved all MLKL_NTD domain-containing (CDD cd21037) proteins and DUF1221 domain-containing proteins from Poaceae and Arabidopsis in the Interpro database ( https://www.ebi.ac.uk/interpro ). Subsequently we performed a BLASTP analysis with the MLKL_NTD domain of Pm13 across the whole-genomes of T. aestivum (cv. Chinese Spring), T. urartu (cv. G1812), Ae. tauschii (cv. AL8/78), T. turgidum dicoccoides (cv. Zavitan), T. turgidum durum (cv. Svevo), Hordeum vulgare (cv. Morex), Secale cereale (cv. Weining), Thinopyrum elongatum (cv. D-3458), and five Sitopsis species of Aegilops genus ( Ae. bicornis cv. TB01, Ae. longissima cv. TL05, Ae. searsii cv. TE01, Ae. sharonensis cv. TH02, and Ae. speltoides cv. TS01) at WheatOmics ( http://wheatomics.sdau.edu.cn/ ) [96] with the default setting. The MLKL_NTD domains of the corresponding proteins in the output from WheatOmics were verified in the NCBI Conserved Domain Search ( https://www.ncbi.nlm.nih.gov/Structure/cdd/wrpsb.cgi ). The phylogenetic trees were constructed using the neighbor-joining method in MEGA7 [97] and drawn with iTOL ( https://itol.embl.de/ ). Collinearity analysis among different species or subgenomes was performed using the online tool Triticeae-GeneTribe with the default parameters [98] . Validation of Pm13 functional molecular markers CS, CS- Ae. longissima 3S l #2(3B) disomic substitution line TA3575, CS- Ae. longissima T3S l #1S-3BS.3BL recombinant R1B, CS- Ae. longissima T3S l #1S-3DS.3DL recombinant R2B, CS- Ae. longissima T3S l #2S-3BS.3BL recombinant W12-3 with tiny 3S l #2 segment harboring Pm13 developed in this study and 180 wheat lines (Supplementary Data 15 ) were used to validate Pm13 functional molecular markers AelMLKL-1 and AelMLKL-8. Genomic DNAs of leaf tissues from these plant materials were extracted using cetyltrimethylammonium bromide (CTAB) method. PCRs were performed in 15 µL volumes containing 7.5 µL 2 × Es Taq MasterMix (CWBIO, Beijing, China), 1.0 µL of each primer (5.0 µmol/L), 2.0 µL template gDNA (100 ng/µL) and 3.5 µL ddH 2 O. The PCR thermocycling conditions were initial denature at 95 °C for 5 min, 35 cycles of 95 °C for 30 s, 58 °C for 30 s, and 72 °C for 1 min, followed by a final extension at 72 °C for 10 min. PCR products were separated via gel-electrophoresis on a 2.0% agarose gel stained with ethidium bromide and visualized by UV light. Reporting summary Further information on research design is available in the Nature Portfolio Reporting Summary linked to this article.